Expansion of the mutually exclusive spliced exome inDrosophila Mutually exclusive splicing is an important mechanism in a wide range of eukaryotic branches to expand proteome diversity, but the extent of its distribution within a single species and its evolutionary conservation is unknown. Here we present a genome-wide analysis of mutually exclusive spliced exons (MXEs) in Drosophila melanogaster at unprecedented depth. Most of the new MXE candidates are supported by evolutionary conservation, transcriptome data analysis and identification of competing RNA secondary structural elements. The enrichment of the genes with MXEs in transmembrane transporters and ion channel activity is consistent with findings in humans, although the MXEs appeared independently and in non-homologous genes, supporting the idea of a universal benefit of adapting ion channel and receptor properties by tandem exon duplications. The comparison of the mutually exclusive spliced exomes within the Drosophila clade shows high numbers of MXE gain and loss events, suggesting a role of these processes in speciation. Alternative processing of primary RNA transcripts is an important driver of increased proteome diversity and regulated gene expression in eukaryotes. Alternative splicing has been reported for alveolates [1] , [2] and stramenopiles [3] , green algae [4] and plants [5] , the cryptophyte Guillardia theta and the chlorarachniophyte Bigelowiella natans [6] , fungi [7] and metazoa [8] , [9] , [10] , and has therefore been an essential characteristic of the last common ancestor of the eukaryotes. The prevalence of the splice types and the overall number of events strongly differ between branches and species. For instance, intron retention is the preferred type in fungi and plants, whereas most mammalian isoforms are produced by exon skipping. A particularly interesting type of generating alternative transcripts is mutually exclusive splicing, which means that exons of clusters of the internal exons are spliced in a mutually exclusive manner. For example, the Drosophila Down Syndrome Cell Adhesion Molecule ( Dscam ) gene contains 95 mutually exclusive spliced exons (MXEs) representing the most extensively alternatively spliced gene known [11] , [12] . Mutations in MXEs and regions regulating their splicing cause human diseases like the Timothy syndrome [13] , cardiomyopathy [14] or cancer [15] , [16] . Mutually exclusive splicing has been shown to be regulated by competing RNA secondary structures [11] , [17] , [18] . Evidence for alternative splicing has mainly been derived by complementary DNA and transcriptome sequencing. However, isoforms might be expressed infrequently in very few tissues or might have very short half-lives hindering their identification with experimental methods, although huge efforts were undertaken to determine the complete transcriptomes of human and model organisms [8] , [9] , [10] , [19] , [20] . Computational approaches integrating biological knowledge could fill this gap. The annotation of the D. melanogaster genome is in a particularly advanced state, owing to protein purification [21] , expressed sequence tag (EST) sequencing [22] , [23] , transcriptome sequencing [10] , DNA microarray studies [24] , [25] , [26] , proteomics studies [19] and whole-genome sequencing of closely related Drosophila species [27] , [28] , [29] . Therefore, it provides a good platform for assessing new methods and validating predictions thereof. Despite the vast amount of these high-throughput data, our understanding of MXE splicing in a genome-wide context is limited. Little is known about the evolution of the mutually exclusive spliced exome. Here we determine the mutually exclusive spliced exome of D. melanogaster with the help of an in silico prediction pipeline [30] and provide evidence for newly predicted MXE candidates by experimental data and evolutionary conservation. We report on the continuous rapid gain and loss of MXEs across 12 Drosophila species. Characteristics of MXEs MXEs have to fulfill the following essential preconditions: They need to be arranged next to each other in clusters, the reading frames must be preserved and the splice site patterns, such as GT–AG, GC–AG or AT–AC, must be compatible for flanking constitutive exons and the MXEs. In addition, we expect these exons to have a similar length, if they code for the same region in the tertiary structure of the encoded protein. Thus, length differences are only possible in some loop regions to not disturb the overall protein structure. For the same reason and as MXEs likely evolved from exon duplication events, we expect high sequence similarity between those exons, especially in the slower evolving protein sequences. Higher sequence conservation between MXEs compared with skipped exons has already been observed for human, indicating their unusual biological importance [8] . Discovery of MXEs To assess the predictive power of these criteria, we analysed all annotated internal MXEs of D. melanogaster (Flybase r5.36; Fig. 1 ). The number of MXEs was evaluated as a function of sequence similarity and maximal length difference, whereas the minimal length of the exons was set to 15 aa ( Supplementary Fig. S1 ). The Drosophila genome contains 60 genes, with 261 annotated internal MXEs of which 251 exons (96.2%) in 55 genes (92%) have length differences of <25 aa (239 have length differences of <10 aa; Supplementary Fig. S2 ), and 234 exons (89.7%) have similarity scores of >1% within the respective clusters ( Supplementary Fig. S3 ). Using these parameters, we would predict 744 genes to encode 3,583 internal MXEs. However, already at more stringent values false-positive candidates are predicted, such as an additional exon candidate for the first cluster of MXEs in the well-studied muscle myosin heavy chain gene ( Mhc ; length difference of 1 and score of 10.4%). Therefore, we decided to use relatively stringent parameters for the analysis, a maximum length difference of 20 aa and a similarity score of 15%, to avoid the incorporation of many false positives, while being aware that we will miss some of the most divergent cases ( Supplementary Fig. S4 ). Under these criteria, 43 genes (71.7%) encode 218 annotated internal MXEs (83.5% sensitivity) and additional 201 high-confidence MXE candidates were predicted, of which 44 are completely new exons in 40 genes ( Fig. 1a and Supplementary Figs S5–S7 ). To exclude that the determined characteristics are Drosophila -specific, we also analysed the annotated mutually exclusive exomes of Homo sapiens (NCBI release 37.3), Caenorhabditis elegans (WormBase release WS230) and Arabidopsis thaliana (TAIR release 167; Supplementary Figs S1–S3 ). At a length difference of 20 aa and a similarity score of 15%, 58% (84 of 144) of human MXEs and 54% (19 of 35) of worm MXEs could be reconstructed, while the At annotation (14 MXEs) does not contain MXEs matching our criteria. This analysis indicates that we have determined species-independent parameters to predict MXE candidates. The high sensitivity of the method implies that most of the new MXE candidates are real exons, which have escaped experimental detection so far. 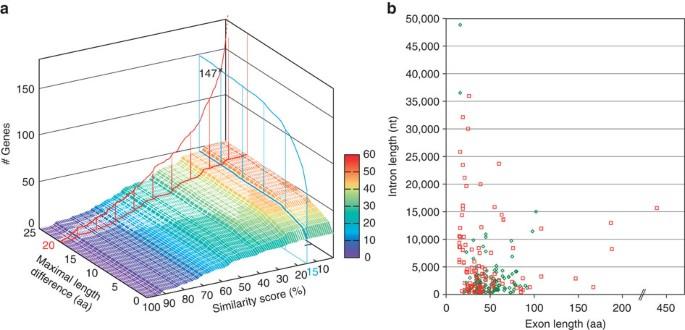Figure 1: Assessing annotated and predicted MXEs. (a) Dependence of the number of genes containing internal MXEs on the maximal length difference and similarity between search exon and MXE candidate. The coloured grid denotes the number of genes with MXEs as annotated in FlyBase r5.36 that were also predicted by WebScipio. The red and blue lines mark the number of genes containing predicted MXE candidates at the maximal length difference of 20 amino acids and at the minimal similarity score of 15%, respectively. (b) Scatter plot of the internal MXE candidates. Green, annotated in r5.36; red, predicted MXEs. Figure 1: Assessing annotated and predicted MXEs. ( a ) Dependence of the number of genes containing internal MXEs on the maximal length difference and similarity between search exon and MXE candidate. The coloured grid denotes the number of genes with MXEs as annotated in FlyBase r5.36 that were also predicted by WebScipio. The red and blue lines mark the number of genes containing predicted MXE candidates at the maximal length difference of 20 amino acids and at the minimal similarity score of 15%, respectively. ( b ) Scatter plot of the internal MXE candidates. Green, annotated in r5.36; red, predicted MXEs. Full size image Very short exons and very long introns increase the chances of predicting false candidates. To exclude potential mispredictions, we analysed the exon lengths of annotated MXEs and the lengths of introns surrounding them ( Fig. 1b ). Exon lengths of MXEs are at least 15 residues (also found for human and Caenorhabditis MXEs, Supplementary Fig. S8 ). The introns surrounding annotated MXEs vary from 50 to 50,000 bp ( Fig. 1b and Supplementary Fig. S9 ). Although most introns range up to 5,000 bp, we therefore cannot assume that potential MXE candidates in longer introns are false predictions ( Supplementary Fig. S10 ). MXE candidates, which are also conserved in other arthropods, were found, for example, in very long introns of the nAcRalpha-80B and bruno-3 genes ( Supplementary Fig. S9 ). Characteristics of MXEs To identify further parameters characterizing MXEs and to ensure that the predicted MXEs have the same features as the already annotated MXEs, we analysed these exons in comparison with all exons in the genome and the subset of constitutive exons matching the criteria of MXEs. The comparison of the exon and intron lengths did not reveal any distinctive features ( Supplementary Figs S11–S14 ). In terms of GC content, the annotated MXEs, which we could not reconstruct, and the constitutive exons, which match the criteria for MXEs, have higher GC contents than the MXEs, which we could reconstruct and which we predict ( Supplementary Fig. S15 ). However, the distribution of the GC content is very broad for all types of exons ranging from 30 to 65%, so that this cannot be taken as a criterion for exclusion. On the basis of the FlyBase annotation, MXEs are found in longer genes, and this is also true for the predicted MXE candidates ( Supplementary Fig. S16 ). The codon usage is almost identical in all types of exons, except for a considerably higher content of alanines (GCC codon) and glutamines (CAA and CAG) in the MXEs, which were annotated in FlyBase but which we could not reconstruct ( Supplementary Fig. S17 ). The 5′-splice junctions of constitutive and MXEs are also slightly different, the latter having a higher priority for G in the −1 and a lower priority for GT in the +5 and +6 positions ( Supplementary Figs S18 and S19 ). Analysis of the start and end phases of the exons showed that the percentage of symmetric exons is a bit higher for the predicted and not annotated MXEs (51%) compared with that of the already annotated but not predicted MXEs (26%, Supplementary Fig. S20 ). This might indicate that some of the predicted MXEs might rather be spliced as constitutive or differentially included exons. Altogether, further discriminative features between MXEs and constitutive exons to be included in the search parameters could not be determined. MXEs versus constitutive and differentially included exons The number of false positives and true negatives could only be determined if an absolutely correct annotation of all genes were available. Although such a data set is missing, we tried to estimate the number of false-positive predictions by searching for constitutive and differentially included exons that match the criteria of MXEs. Of the 60,401 exons annotated as constitutive or differentially included exons in the D. melanogaster genome, only 169 exons (0.28%) in 46 genes matched these criteria. Several of these exons are even annotated as MXEs in the latest FlyBase release based on RNA-Seq evidence, including a cluster of MXEs in the βTub97EF gene, the Lipophorin receptor 1 gene and the nicotinic Acetylcholine Receptor α 30D gene ( Supplementary Fig. S21 ). This demonstrates that only a minor part of all internal exons matching the characteristics of MXEs is spliced constitutively, and we conclude that most of the new MXE candidates will be spliced in a mutually exclusive way. The mutually exclusive spliced exome of D. melanogaster To characterize the mutually exclusive spliced exome, we identified 1,297 exons that are mutually exclusive in annotated isoforms of the same gene ( Supplementary Tables S1 and S2 ). Of these, 291 had similar length and sequence, including 218 internal MXEs. We predicted 539 exons of similar length and sequence that could be spliced in a mutually exclusive way (two times the annotated exons; Fig. 2 , Supplementary Figs S22 and S23 , and Supplementary Data 1 and 2 ). Four hundred and nineteen of the MXE candidates were internal, including 218 of the already annotated MXEs. Evidence for the predicted MXE candidates was obtained through additional data ( Fig. 2 and Supplementary Data 3 ): (A) Mapping of EST and RNA-Seq data. (B) Conservation of the MXE candidates in other arthropods. For this purpose, we identified the homologues to the D. melanogaster genes in 11 sequenced Drosophila species, as well as in Anopheles gambiae , Aedes aegypti , Atta cephalotes , Apis mellifera , Tribolium castaneum , Pediculus humanus corporis and Daphnia pulex , and predicted MXE candidates in the homologues using the same pipeline as for D. melanogaster . (C) Ab initio prediction of exonic regions in the respective introns using AUGUSTUS [31] . (D) Identification of competing RNA secondary structures. Of the internal MXEs, 57% were supported by multiple data types, 21% were supported by EST data. Of the 44 newly predicted internal MXEs, 8 were supported by EST and/or RNA-Seq data. Of the annotated and reconstructed internal MXEs, and of the total predicted internal MXEs, 94.5% and 76.6%, respectively, are evolutionarily conserved in at least 1 of the 18 further analysed species. In total, only 120 cases of terminal MXEs have been identified with similar length and sequence. These exons are, however, spliced by alternative cleavage and polyadenylation and/or alternative promotor usage, and represent only 73 (7.0%) of the annotated 1,036 terminal MXEs. As many of these terminal MXE candidates belong to predicted genes, which are not yet supported by full-length cDNA or RNA-Seq data, some might turn to internal exons if further 5′ and 3′ exons are identified. 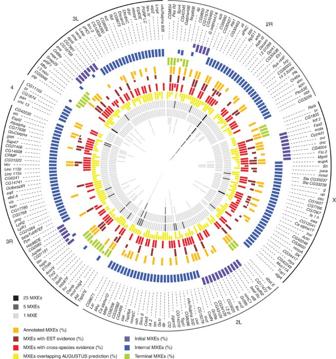Figure 2:The mutually exclusive exome ofDrosophila melanogaster. All genes containing predicted MXEs are listed. The grey bars denote the number of MXEs predicted for each gene and the coloured bars display the evidence by various criteria, in per cent. Figure 2: The mutually exclusive exome of Drosophila melanogaster . All genes containing predicted MXEs are listed. The grey bars denote the number of MXEs predicted for each gene and the coloured bars display the evidence by various criteria, in per cent. Full size image Examples of supported new MXE candidates The genes containing annotated or predicted MXEs are almost evenly spread on all chromosomes ( Fig. 2 and Supplementary Data 3 ). Seventy-five per cent of them are named and have at least one functional study linked in FlyBase. As an example, the new gene model of the vibrator ( vib ) gene coding for a phosphatidylinositol transfer protein contains a cluster of MXEs, which was not known in r5.36 but is supported by EST and RNA-Seq data, and is included in the latest release r5.48 ( Fig. 3a ; for the complete list of new MXE candidates not included in r5.36 but in r5.48, see Supplementary Fig. S22 ). Examples of new clusters of MXEs in well-known genes that are not included in r5.48 include the Shaker ( Sh ) gene, in which the cluster is conserved in all arthropod species analysed and of which the 3′-end of the new MXE candidate is supported by RNA-Seq data, and the nicotinic Acetylcholine Receptor α 80B ( nAcRalpha-80B ) gene, in which the cluster is conserved from Daphnia to mosquitoes and Drosophila but not yet supported by experimental data ( Fig. 3a ; for the complete list of new MXE candidates not included in r5.48, see Supplementary Fig. S23 ). The evolutionary conservation provides high confidence to the new MXE candidates. The missing experimental support indicates that the new MXE candidates either represent low-abundance isoforms or variants restricted to very specific cell types and developmental stages, which were not yet covered by the RNA-Seq read depth and tissue selection [8] , [10] . For instance, the expression of an MXE isoform of the human calcium channel Ca V 2.2 is restricted exclusively to nociceptive neurons of dorsal root ganglia [32] . However, the MXE expression could also be regulated differently in other individuals than in the sequenced fly and in other species. Interindividual variation has been found to be very common in humans, although still less frequent than variation between tissues [8] , but has not yet been shown for Drosophila . 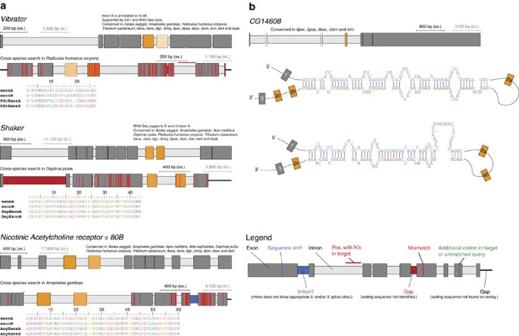Figure 3: Examples of new MXE candidates. (a) Exon–intron gene structures of example genes containing newly predicted internal MXEs. The isoforms of thevibratorgene are annotated in r5.48 and are supported by cDNA and RNA-Seq, theshakergene splice variants are not annotated but supported by RNA-Seq, and the MXE candidate of thenicotinic Acetylcholine Receptor α 80Bis not experimentally supported yet. (b) Exon–intron gene structure of theCG14608gene containing two newly predicted internal MXEs that are supported by evidence through competing RNA secondary structures. All transcripts are represented 5′ to 3′. The colour coding is explained in the legend and applies to all gene structure figures. Coloured big bars represent mutually exclusive exons. The darkest coloured bar is the exon that was included in the query sequence, whereas the lighter coloured bars represent identified MXEs. The higher the similarity between the candidate and the query exon, the darker the colour of the candidate (100% identity would result in the same colour). The opacity of the colours of each alternative exon corresponds to the alignment score of the alternative exon to the original one. Figure 3: Examples of new MXE candidates. ( a ) Exon–intron gene structures of example genes containing newly predicted internal MXEs. The isoforms of the vibrator gene are annotated in r5.48 and are supported by cDNA and RNA-Seq, the shaker gene splice variants are not annotated but supported by RNA-Seq, and the MXE candidate of the nicotinic Acetylcholine Receptor α 80B is not experimentally supported yet. ( b ) Exon–intron gene structure of the CG14608 gene containing two newly predicted internal MXEs that are supported by evidence through competing RNA secondary structures. All transcripts are represented 5′ to 3′. The colour coding is explained in the legend and applies to all gene structure figures. Coloured big bars represent mutually exclusive exons. The darkest coloured bar is the exon that was included in the query sequence, whereas the lighter coloured bars represent identified MXEs. The higher the similarity between the candidate and the query exon, the darker the colour of the candidate (100% identity would result in the same colour). The opacity of the colours of each alternative exon corresponds to the alignment score of the alternative exon to the original one. Full size image Alternative splicing of the Mhc and the Dscam genes in arthropods has been shown to be regulated by RNA secondary structures [18] , [33] . Docking sites (acceptor sequences) have been identified in the introns in front or behind the cluster of MXEs to which only one of the selector sequences downstream or upstream of each MXE, respectively, can bind at a time, forming conserved base-pairing interactions. Although such sites have only been found for some of the MXE clusters in the 14-3-3ζ , the Mhc and the Dscam genes, this mechanism might also regulate the splicing of other MXE clusters. We searched for complementing sequences in all predicted clusters of MXEs and found favourable sites in many of the annotated clusters. The CG14608 gene exemplifies a predicted cluster of MXEs, for which RNA-Seq evidence is not available, but which is supported by cross-species evidence and by competing RNA secondary structure prediction ( Fig. 3b and Supplementary Fig. S24 ). Functional analysis of the genes containing MXEs To analyse the conservation pattern of the genes containing MXEs with respect to their involvement in biological processes, we performed a Gene Ontology (GO) analysis [34] . Surprisingly, the genes with annotated and reconstructed MXEs, as well as the genes with predicted but not annotated MXEs, both display strong enrichment in transmembrane transporter and ion channel activity, and plasma membrane localization ( Supplementary Figs S25 and S26 ). It has been shown for human that genes with MXEs are more often involved in regulating highly tissue-specific functions than genes with spliced exons, and that these genes are enriched in cell communication and signal trunsduction [8] . Tandem exon duplications have occurred, for example, in many of the human, C. elegans and Drosophila ion channels, in both voltage- and calcium-gated types [35] , and in glycine, glutamate and nicotinic acetylcholine receptors [35] , [36] . However, the exons duplicated independently, and not only in homologous but also non-homologous families. It has therefore been suggested that exon duplications provide a general benefit of adapting ion channel and receptor functions compared with gene duplications [35] . Although not shown yet, MXEs in these genes are probably a common property of all metazoans. The GO analysis of the new Drosophila MXE candidates showing a similar enrichment in biological processes as in annotated genes indicates that the recent experimental approaches were not yet exhaustive enough and that our approach is a valuable complement to unveil the mutually exclusive exome of a species. Evolution of the MX spliced exome in 12 Drosophila It is well known that the clusters of MXEs are highly conserved, for example, in the Drosophila Mhc genes [37] , whereas some variability has been observed for the Dscam genes [11] , [30] . To determine the extent of conservation within the Drosophila MXEs, we compared the data from D. melanogaster (dmel) with the reconstructed corresponding exomes of 11 further Drosophila species ( Fig. 4a ). In total, 2,640 clusters were identified, most of which are shared among several species, resulting in 770 unique clusters. The genomes of dsim, dsec and dper are less complete than the other assemblies and were, therefore, analysed in groups, resulting in seven Drosophila species or species groups ( Fig. 4a ). Surprisingly, many of the clusters are unique to one of these groups, such as 164 clusters within the Drosophila subgenus group (dvir, dmoj and dgri) or 95 clusters within the obscura group (dpse and dper). Only 68 clusters are conserved in all 12 species (115 in the seven groups). Thirty-six clusters are missing in only 1 of the species and 16 clusters are absent in any 2 species. The alternative exons of these clusters could have been lost in these species because of a single, independent exon-loss event, or have not been detected. Potential reasons for the latter can be gaps in the assemblies, leading to the absence of entire and partial genes or single exons, and exon sequence divergence, leading to their exclusion under the given cutoff values. However, most clusters are shared by at least two species or species groups, and it is very unlikely that assembly gaps are present in independent genomes at exactly the same region in all the other species. Examples are the Cacophony gene, for which an additional conserved cluster of MXEs was identified in dwil, dgri, dvir and all other arthropods analysed that has, however, been lost in dmel and the other Drosophila species ( Fig. 4b ), and the Ras opposite ( Rop ) gene, which is a single-exon gene in dmel, dere, dsec and dyak, but a multi-exon gene containing a conserved cluster of MXEs in dwil, dgri, dper, dvir and the other arthropods ( Fig. 4c ). The predicted clusters of MXEs, therefore, represent MXEs of which the alternative exons have been lost in certain species, or exons that have been gained at a certain step in Drosophila evolution. To determine exon gain and loss during the evolution of the Drosophila species, we counted these events based on maximum parsimony requiring the least exon-loss events ( Fig. 5 ). The last common ancestor of the Drosophila species contained at least 186 clusters of MXEs (24.2% of all unique clusters). Four hundred and fifty-six clusters (59.2%) are unique to any of the Drosophila species and 111 clusters (14.4%) have been gained in certain branches. 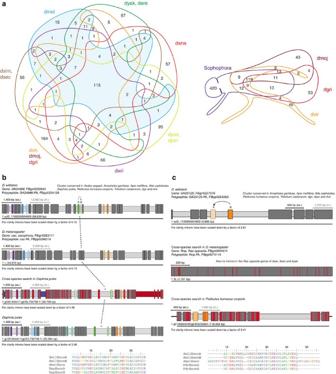Figure 4: Evolution of mutually exclusive splicing clusters. (a) The Venn diagrams48show the number of clusters of MXEs shared between species and subsets of species groups. Species abbreviations areD. simulans(dsim),D. sechellia(dsec),D. melanogaster(dmel),D. yakuba(dyak),D. erecta(dere),D. ananassae(dana),D. pseudoobscura(dpse),D. persimilis(dper),D. willistoni(dwil), which are all part of the Sophophora branch, andD. virilis(dvir),D. mojavensis(dmoj) andD. grimshawi(dgri). (b) The gene structure of theD. melanogaster Cacophonygene is shown in comparison with its homologues inD. willistoniandDaphnia pulex. TheD. melanogastergene contains three clusters of MXEs. A forth cluster is present inD. willistoni,Daphniaand in other insects that had been lost inD. melanogaster. The respective corresponding exons are marked by dotted lines, and their sequences are shown in the alignment. (c) The gene structure of theD. melanogaster Ras oppositegene is shown in comparison with its homologues inD. willistoniandPediculus humans corporis. TheD. melanogastergene consists of a single exon as do the homologues in dere, dsec and dyak. The introns of this gene must have been lost in the ancestor of the melanogaster subgroup branch. In contrast, theRas oppositegene inD. willistoniis a multi-exon gene and contains a cluster of MXEs. This cluster of MXEs is also found inPediculusand most of the other analysed insect species. The sequences of the MXEs as well as the corresponding region in theD. melanogasterprotein are shown in the alignment. All transcripts inbandcare represented 5′ to 3′. Coloured big bars represent mutually exclusive exons. The darkest coloured bar is the exon that was included in the query sequence, whereas the lighter coloured bars represent identified MXEs. The higher the similarity between the candidate and the query exon, the darker the colour of the candidate (100% identity would result in the same color). The opacity of the colours of each alternative exon corresponds to the alignment score of the alternative exon to the original one. Figure 4: Evolution of mutually exclusive splicing clusters. ( a ) The Venn diagrams [48] show the number of clusters of MXEs shared between species and subsets of species groups. Species abbreviations are D. simulans (dsim), D. sechellia (dsec), D. melanogaster (dmel), D. yakuba (dyak), D. erecta (dere), D. ananassae (dana), D. pseudoobscura (dpse), D. persimilis (dper), D. willistoni (dwil), which are all part of the Sophophora branch, and D. virilis (dvir), D. mojavensis (dmoj) and D. grimshawi (dgri). ( b ) The gene structure of the D. melanogaster Cacophony gene is shown in comparison with its homologues in D. willistoni and Daphnia pulex . The D. melanogaster gene contains three clusters of MXEs. A forth cluster is present in D. willistoni , Daphnia and in other insects that had been lost in D. melanogaster . The respective corresponding exons are marked by dotted lines, and their sequences are shown in the alignment. ( c ) The gene structure of the D. melanogaster Ras opposite gene is shown in comparison with its homologues in D. willistoni and Pediculus humans corporis . The D. melanogaster gene consists of a single exon as do the homologues in dere, dsec and dyak. The introns of this gene must have been lost in the ancestor of the melanogaster subgroup branch. In contrast, the Ras opposite gene in D. willistoni is a multi-exon gene and contains a cluster of MXEs. This cluster of MXEs is also found in Pediculus and most of the other analysed insect species. The sequences of the MXEs as well as the corresponding region in the D. melanogaster protein are shown in the alignment. All transcripts in b and c are represented 5′ to 3′. Coloured big bars represent mutually exclusive exons. The darkest coloured bar is the exon that was included in the query sequence, whereas the lighter coloured bars represent identified MXEs. The higher the similarity between the candidate and the query exon, the darker the colour of the candidate (100% identity would result in the same color). The opacity of the colours of each alternative exon corresponds to the alignment score of the alternative exon to the original one. 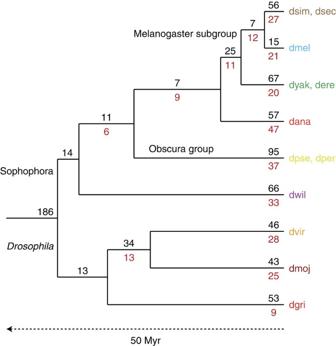Figure 5: The gain and loss of clusters of MXEs. The gain and loss of clusters of MXEs plotted onto the evolutionary tree of theDrosophilaspecies (black and red numbers, respectively). Species abbreviations areD. simulans(dsim),D. sechellia(dsec),D. melanogaster(dmel),D. yakuba(dyak),D. erecta(dere),D. ananassae(dana),D. pseudoobscura(dpse),D. persimilis(dper) andD. willistoni(dwil), which are all part of the Sophophora branch, andD. virilis(dvir),D. mojavensis(dmoj) andD. grimshawi(dgri). Full size image Figure 5: The gain and loss of clusters of MXEs. The gain and loss of clusters of MXEs plotted onto the evolutionary tree of the Drosophila species (black and red numbers, respectively). Species abbreviations are D. simulans (dsim), D. sechellia (dsec), D. melanogaster (dmel), D. yakuba (dyak), D. erecta (dere), D. ananassae (dana), D. pseudoobscura (dpse), D. persimilis (dper) and D. willistoni (dwil), which are all part of the Sophophora branch, and D. virilis (dvir), D. mojavensis (dmoj) and D. grimshawi (dgri). Full size image The presence of a large subset of MXEs in at least two Drosophila species, which are not closest relatives, implies frequent MXE gain and loss events during insect evolution. Compared with the conserved set of MXEs, the number of species-specific gains and losses is striking. This pattern suggests that exon duplication leading to MXEs is a very active process that might contribute to speciation. Similarly, changes in the alternative splicing patterns in vertebrates have been found to contribute more to vertebrate speciation and tissue specification than gene expression programmes do [38] , [39] . Exon duplication is a very convenient way to increase protein diversity by only modulating a domain or subdomain function. In contrast to gene duplications, the gene dosage is most likely not altered in genes after exon duplication eliminating the need for a relaxed selection against degenerative mutations. Thus, exon duplicates are immediately subject to stabilizing selection and could improve different functions of the original exons. Our analysis of the mutually exclusive exome of D. melanogaster considerably increased the number of mutually exclusive splicing events. Specifically, we have identified two times more internal MXE candidates than that already annotated, of which almost 80% are supported by evolutionary conservation or experimental transcript data. This number is surprising given the enormous and long-standing efforts in annotating the D. melanogaster genome. However, annotation is a continuous process and even a recent exhaustive exploration of the developmental transcriptome of D. melanogaster using RNA-Seq, tiling microarrays and cDNA sequencing failed to detect expression of 12% of the known genes, although the coverage of the genome and transcriptome were 1,200- and 5,900-fold, respectively [10] . This is consistent with a recent proteomics study showing that MXEs are highly underrepresented in RNA-Seq data [19] . Because of the tight cut-offs of our analysis, we are sure that many more MXEs can be identified through manual investigation of the unexplored data. Here we provide an important step in completing the D. melanogaster genome annotation and a valuable resource for further studies. The method has also been applied to the human, C. elegans and A. thaliana genomes for comparison. In all genomes, many more MXE candidates could be identified than the ones annotated, although MXE splicing is not as prevalent as in Drosophila . However, the water flea Daphnia pulex has two to three times more genes with clusters of MXEs than that in D. melanogaster , and we are sure that this particular alternative splice type is even more widespread in other species. Our method provides a straightforward way to analyse other genomes in the future, including resolving artificial fusions of tandemly arrayed gene duplicates and candidates for trans -splicing. Given the suggested unusual biological importance of the MXEs in human [8] compared with skipped exons, the rapid evolution of the mutually exclusive exomes of the 12 Drosophila species is all the more surprising. It indicates an important role of the corresponding genes and the necessity to conserve the overall shape of the proteins while creating diversity in restricted regions. Reconstruction of gene structures Genome assemblies and annotated proteins for the Drosophila species were obtained from FlyBase [40] (r5.36 for D. melanogaster , r 1.2 for D. virilis , r 2.25 for D. pseudoobscura and r 1.3 for all other Drosophila species), for Caenorhabditis elegans from WormBase [41] (WS 230), for Arabidopsis thaliana from TAIR [42] (v. 10) and for human from GenBank (v. 37.3). EST data were downloaded from GenBank. More details about the data sets are given in Supplementary Table S3 . The gene structures for the annotated proteins were reconstructed with Scipio [43] using standard parameters, except max_mismatch=7, region_size=20,000 (50,000 for D. melanogaster ), single_target_hits, max_move_exon=10, gap_to_close=0, blat_oneoff=false, blat_score=15, blat_identity=54, exhaust_align_size=20,000 and exhaust_gap_size=50. Scipio starts with a blat_tilesize of 7 and reduces this step by step to 4, if parts of the protein sequence could not be found. All parameters are less stringent than default parameters to increase the chance to reconstruct all genes automatically. The region_size, which determines the number of up- and downstream nucleotides added to the gene sequence, has been increased to allow searching for 5′ and 3′ candidates of MXEs. Predicting MXEs MXEs were predicted in the reconstructed genes using the algorithm implemented in WebScipio [30] with a minor modification favouring GT–AG splice junctions over the other possible splice sites (GC–AG and GG–AG) if several overlapping candidates existed. As initial parameters for MXE candidate predictions in D. melanogaster , we set the length difference to 25 aa, the minimum score to 1 and the minimum exon length to 1. For all other species, the parameters were length difference=20, minimum score=10 and minimum exon length=10. MXE candidates were searched for all exons in all introns, and up- and downstream regions. Candidates for 5′-exons of genes were expected to start with a methionine, and candidates for 3′-exons of genes were expected to end with a stop codon. Obtaining evidence for MXE candidates Ab initio exon prediction was done with AUGUSTUS using default parameters to find alternative splice forms and the feature set for D. melanogaster . Cross-species searches and mapping of EST data were done with WebScipio with same parameters as for gene reconstructions, except min_identity=60, max_mismatch=0 (allow any number of mismatches), gap_to_close=10, min_intron_length=35, blat_tilesize=6 and blat_oneoff=true. MXE candidates in cross-species gene reconstructions were searched with length difference=20, minimum score=15 and minimum exon length=15, for all exons in all introns but not in up- and downstream regions. Binding windows for competing intron RNA secondary structures were predicted for all candidate clusters of MXEs using the SeqAn [44] package. The identified binding windows of all homologous genes were aligned using MUSCLE [45] and the RNA secondary structures predicted by RNAalifold (ViennaRNA package) [46] . The GO enrichment analysis was done with AmiGO [47] . All data can be searched, filtered and browsed at Kassiopeia ( www.motorprotein.de/kassiopeia ). For upload into the FlyBase genome browser, a GFF file containing the complete gene structures of the genes that include new MXEs, and a GFF file containing only the clusters of MXE candidates are available as Supplementary Data 1 and 2 . Accession code: Sequences for spliced exons have been deposited in the Kassiopeia database under accession numbers dmel00001 to dmel00539. How to cite this article: Hatje, K. et al. Expansion of the mutually exclusive spliced exome in Drosophila . Nat. Commun. 4:2460 doi: 10.1038/ncomms3460 (2013).